Diastereo- and enantioselective [3 + 3] cycloaddition of spirocyclopropyl oxindoles using both aldonitrones and ketonitrones Optically active spirocyclic compounds play an important role in drug discovery, and new synthetic strategies for the efficient generation of spiro stereocenters are in much demand. Here we report a catalytic enantioselective cycloaddition using spirocyclic donor–acceptor cyclopropanes as a promising approach for the generation of spiro stereocenters. A diastereo- and enantioselective [3 + 3] cycloaddition of spirocyclopropyl oxindoles with both aldonitrones and ketonitrones is developed. The key to reaction development is the activation of spirocyclopropyl oxindoles by a suitable electron-withdrawing N -protecting group. This activation approach offers the promise of a general solution to enable spirocyclopropyl oxindoles as synthons for catalytic enantioselective synthesis of spirocyclic oxindoles featuring a C3 spiro stereocenter, a prominent structural motif in drugs and pharmaceutically active compounds. This protocol also constitutes the catalytic enantioselective reaction using unactivated achiral ketonitrones to construct tetrasubstituted carbon stereocenters. To enhance the reward in modern probe- and drug-discovery programs, there is a vast demand for synthetic libraries of optically active compounds recapitulating the structural features of privileged scaffolds that widely present in natural products, drugs, and pharmaceutically active compounds [1] . In this context, spirocyclic compounds have found ever-increasing utilization in drug discovery, because the conformational constraints imposed by a spiro-ring fusion often bring about improved biological activities of biomolecules [2] , [3] . Therefore, efficient and enantioselective approaches capable of flexible construction of spiro stereocenters would facilitate the buildup of synthetic libraries of optically active spirocyclic compounds, which will help in the search for new lead candidates. However, the catalytic enantioselective synthesis of spirocyclic sterocenters is still a long-standing challenge in synthetic chemistry, especially when a spiro all-carbon quaternary stereocenter [4] , [5] , [6] is involved. Despite the invention of some elegant protocols [7] , the exploitation of new synthetic routes for the catalytic enantioselective construction of spiro stereocenters is still highly desirable. The catalytic enantioselective cycloaddition reactions of doubly activated donor–acceptor (D−A) cyclopropanes [8] , [9] , [10] , [11] , [12] , [13] with different dienes, 1,3-dipoles or dipolarphiles has been established as a powerful approach for the efficient and diverse synthesis of cyclic compounds [14] , [15] , [16] , [17] , [18] , [19] , [20] , [21] , [22] , [23] , [24] , [25] , [26] , [27] , [28] , [29] , [30] , [31] . However, the application of this strategy to construct spirocycles is largely undeveloped, because known successful protocols all rely on the use of 2-substituted cyclopropane-1,1-dicarboxylates and analogous cyclopropyl diketones (Fig. 1a ) [14] , [15] , [16] , [17] , [18] , [19] , [20] , [21] , [22] , [23] , [24] , [25] , [26] , [27] , [28] , [29] , [30] , [31] . This is possibly because the geminal ester or ketone groups of such cyclopropanes can effectively stabilize the negative charge in the 1,3-zwitterionic intermediates and facilitate the formation of a well-organized catalyst–substrate complex via bidentate chelation, which is often important for enantiocontrol [20] , [21] , [22] , [23] . The use of spirocyclic D−A cyclopropanes for cycloaddition would open new avenues to construct chiral spirocyclic scaffolds (Fig. 1b ); however, although an elegant chiral cyclopropane-based version had been reported [32] , no successful catalytic enantioselective example is currently known [7] , [8] , [9] , [10] , [11] , [12] , [13] . Fig. 1 Enantioselective cycloaddition reactions using D−A cyclopropanes. a Well-established cyclic compounds synthesis. b Undeveloped spiro stereocenter generation compounds synthesis. c Activation of spirocyclopropyl oxindoles for cycloaddition reactions. Donor (D): electron-releasing group; Acceptor (A): electron-withdrawing group (CO 2 R or COR) Full size image For example, spirocyclopropyl oxindoles represent a class of easily available spirocylic D–A cyclopropanes, but the use of such monoactivated D–A cyclopropanes for enantioselective catalysis is largely unexplored [33] . This is surprising, because as early as in 1999, Carreira et al. [34] , [35] , [36] , [37] have successfully utilized unprotected or N -benzyl spirocyclopropyl oxindoles to build up the spiro[pyrrolidine-3,3′-oxindole] ring systems via MgI 2 -catalyzed annulation with imines. Since the absolute configuration and the substituent of the C3 spiro stereocenters of spirocyclic oxindoles greatly influenced the biological activities [38] , [39] , it is of current interest to exploit new catalytic enantioselective methods for the synthesis of spirocyclic oxindoles that are prominent structural motifs in natural products and drugs [38] , [39] , [40] , [41] , [42] , [43] , [44] , [45] , [46] , [47] , [48] , [49] , [50] , [51] , [52] , [53] . While enantioselective cycloaddition using spirocyclopropyl oxindoles as D–A cyclopropanes constitutes a new entry for diverse synthesis of optically active spirocyclic oxindoles, it is difficult to make use of such monoactivated D–A cyclopropanes, for two reasons. First, with only one amide acceptor group, the activity of spirocyclopropyl oxindoles is not high. Second, a high level of transition state organization is difficult to realize simply by monodentate coordination of the amide group to a chiral Lewis acid. To tackle these two challenges, coupled with our interest in oxindole chemistry [54] , [55] , we consider activating spirocyclopropyl oxindoles, easily prepared from olefin cyclopropanation using diazooxindoles [55] , by installing an electron-withdrawing N -protecting group. It may not only improve the stabilization of the negative charge developed at the C3 position of an oxindole via charge separation upon Lewis acid activation, but it may enable the binding of oxindole to chiral catalyst in a bidentate fashion, which is helpful for enantiocontrol. Herein, we demonstrate the power of this approach by a highly diastereo- and enantioselective [3 + 3] cycloaddition of spirocyclopropyl oxindoles and nitrones. Optimization of the reaction conditions A variety of activated spirocyclopropyl oxindoles 1c – e and 2a , with different electron-withdrawing N -protecting groups, were readily prepared in one step from the corresponding unprotected precursor. With these spirocyclic D–A cyclopropanes at hand, we first evaluated their performance in the [3 + 3] cycloaddition reaction using nitrones, because the thus-obtained quaternary spirocyclic oxindoles, merging the structural feature of tetrahydro-1,2-oxazine, are interesting targets for medicinal research. It is worth mentioning that since the pioneering work of Young and Kerr [56] , the [3 + 3] cycloaddition reaction of D–A cyclopropanes and nitrones [56] , [57] , [58] , [59] , [60] has been established as an elegant approach to access tetrahydro-1,2-oxazines, which hold potential as therapeutic agents and as synthons [61] , [62] , [63] . Later, Sibi [18] and Tang [19] independently achieved highly enantioselective versions, which subsequently prompted further studies into catalytic asymmetric synthesis based on D–A cyclopropanes [8] , [9] , [10] , [11] , [12] , [13] , [14] , [15] , [16] , [17] , [18] , [19] , [20] , [21] , [22] , [23] , [24] , [25] , [26] , [27] , [28] , [29] , [30] , [31] . Nevertheless, the use of aliphatic nitrones or ketonitrones for such catalytic enantioselective cycloaddition reactions were undeveloped. 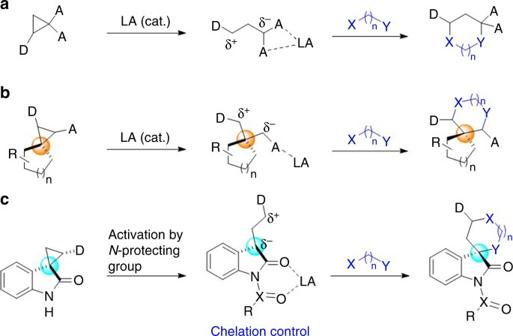Fig. 1 Enantioselective cycloaddition reactions using D−A cyclopropanes.aWell-established cyclic compounds synthesis.bUndeveloped spiro stereocenter generation compounds synthesis.cActivation of spirocyclopropyl oxindoles for cycloaddition reactions. Donor (D): electron-releasing group; Acceptor (A): electron-withdrawing group (CO2R or COR) The N -protecting group of spirocyclopropyl oxindoles in deed plays an important role in securing high reactivity, as shown in Table 1 . All reactions were catalyzed by 10 mol% Ni(OTf) 2 , using 1,2-dichloroethane (DCE) as solvent at 50 °C. For the screening of Lewis acids, see Supplementary Table 1 . Not unexpectedly, the reaction of unprotected oxindole 1a with nitrone 3a resulted in a mess, affording the desired adduct 4a in ca. 30% NMR yield (entry 1, Table 1 ), and no reaction took place in the case of N -benzyl oxindole 1b (entry 2, Table 1 ). In contrast, spirocyclopropyl oxindoles 1c and 1d , activated by a N -acetyl or benzoyl group, exhibited much higher reactivity, giving adducts 4c and 4d in high yields (entries 3–4, Table 1 ). With N - p -tolylsulfonyl group, oxindole 1e also worked well with 3a to give adduct 4e in high yield and dr value (entry 5, Table 1 ). Interestingly, N -diethoxyphosphoryl oxindole 2a showed high activity, and the corresponding reaction could complete within 6 h to give adduct 5a in 95% yield and 20:1 dr (entry 6, Table 1 ). NMR analysis of these adducts 4 and 5 suggested that the N -protecting groups had little influence on the diastereoselectivity; X-ray analysis revealed that the major diastereomer of both N -diethoxyphosphoryl and N -Ts protected adducts have the same relative configuration. 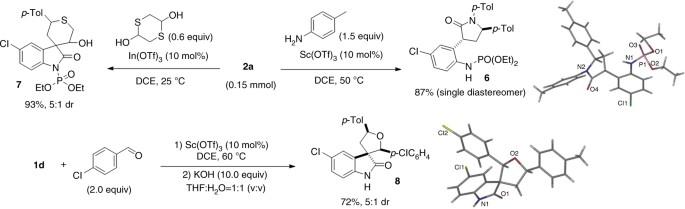Fig. 2 Other typical reactions of the activated spirocyclopropyl oxindoles. Ring opening reaction of2ausingp-toluidine. Cyclization reaction of2awith 1,4-dithiane-2,5-diol. Diploar cycloaddition of1dwith 4-chlorobenzaldehyde, followed by deprotection using KOH. Isolated yield The relative configuration of the minor diastereomer of 4e was also determined by X-ray analysis, which differed from the major diastereomer at the quaternary center of oxindole (see Supplementary Table 2 ). These results strongly support our working hypothesis, namely, that it is possible to activate spirocyclopropyl oxindoles by installing electron-withdrawing N -protecting groups (Fig. 1c ). Table 1 Evaluation of N -withdrawing protection group a Full size table The elaboration of the activated spirocyclopropyl oxindoles Notably, these activated spirocyclopropyl oxindoles could serve as viable synthons for other typical reactions of D–A cyclopropanes as well (Fig. 2 ). For example, N -diethoxyphosphoryl oxindole 2a readily underwent ring-opening/cyclization reaction to give 3,5-disubstituted pyrrolidinone 6 in 87% yield, or reaction with 1,4-dithiane-2,5-diol to afford 7 in 93% yield and 5:1 dr. On the other hand, N -benzoyl oxindole 1d was superior in the [3 + 2] cycloaddition with aldehyde. Because deprotection of the adduct occurred in the reaction course, KOH was added to facilitate the removal of protecting group after cycloaddition finished, furnishing unprotected spirocyclic oxindoles 8 in 72% yield with 5:1 dr. The relative configuration of product 6 and 8 was assigned by X-ray analysis. These results implied it possible to adjust N -electron-withdrawing group to develop new reactions. It should be noted that N -unprotected or N -benzyl analogs 1a and 1b all failed to participate in the three different kinds of reactions, confirming the importance of the activation effect of electron-withdrawing N -protecting group. Fig. 2 Other typical reactions of the activated spirocyclopropyl oxindoles. Ring opening reaction of 2a using p -toluidine. Cyclization reaction of 2a with 1,4-dithiane-2,5-diol. Diploar cycloaddition of 1d with 4-chlorobenzaldehyde, followed by deprotection using KOH. Isolated yield Full size image Substrate scope of the reaction The potential of these activated spirocyclopropyl oxindoles in enantioselective catalysis was further demonstrated by a highly enantioselective [3 + 3] cycloaddition using nitrones. 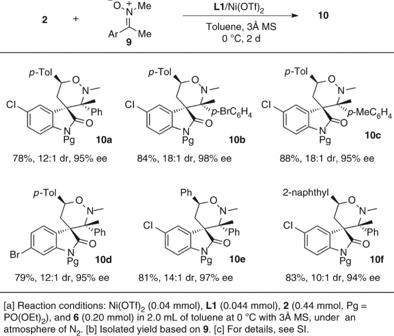Fig. 3 Cycloaddition of spirocyclopropyl oxindoles using ketonitrones. Construction of adjacent quaternary and tetrasubstituted carbon stereocenters The screening of chiral ligands (see Supplementary Table 3 ) revealed that bisoxazoline L 1 [64] /Ni(OTf) 2 complex allowed the synthesis of 5a in 41% yield and 92% ee (entry 1, Table 2 ). Gratifyingly, when the reaction solvent was changed from DCE to THF, both adduct 5a and cyclopropane 2a were obtained with excellent ee values (entries 1–3, Table 2 ). By adjusting the amount of nitrone 3a to 0.55 equiv, adduct 5a was obtained in 49% yield and 97% ee, with 2a recovered in 46% yield and 96% ee (entry 4, Table 2 ). Therefore, the substrate scope was examined using THF as the solvent, in the presence of 10 mol% catalyst L 1 /Ni(OTf) 2 . Table 2 Optimization for enantioselective synthesis Full size table It emerged that both aromatic and aliphatic substituted nitrones were viable substrates for this kinetic resolution, with >20:1 dr values achieved in most cases (Table 3 ). Both electron-deficient and electron-rich α-aryl nitrones 3a – g worked well to afford the desired adducts 5a – g with excellent ee values (entries 1–7, Table 3 ). Nitrones 3h – j with a 2-naphthyl, furyl, or 2-thienyl group all afforded the corresponding adducts 5h – j in excellent yields and ee values (entries 8–10, Table 3 ). In these cases, spirocyclopropyl oxindole 2a was recovered with an excellent ee value and good yield. Interestingly, aliphatic nitrones 3k , l also gave the desired 1,2-oxazine adducts 5k , l in good yields and with >90% ee; cyclopropane 2a , however, was recovered with lower ee values (entries 11–12, Table 3 ). To our knowledge, aliphatic nitrones have not been used for such catalytic enantioselective cycloaddition previously [18] , [19] , [56] , [57] , [58] , [59] , [60] . 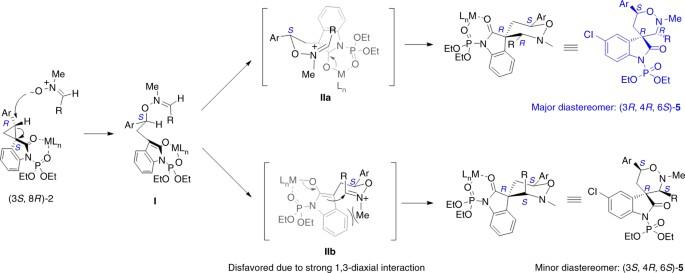Fig. 4 Working model for the observed 3,6-trans selectivity of adducts5. A stepwise annulation mechanism. The favored boat-like transition stateIIais possibly stabilized by the cation–π interaction. The chiral-like transition stateIIbis presumably destabilized by the strong 1,3-diaxial repulsion 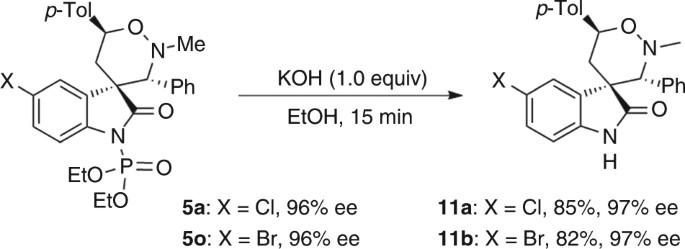Fig. 5 Deprotection of product5aand5o. Reaction conditions:5(0.1 mmol), KOH (1.0 mmol) in 2.0 mL of EtOH at room temperature. Isolated yield Table 3 Scope of different nitrones Full size table On the other hand, the substituents on oxindole framework of cyclopropane 2 were found to have an influence on the reaction outcome (Table 4 ). With electron-withdrawing groups on the C5 or C6 positions, oxindoles 2c – e gave the desired adducts 5n – p in 38–44% yield and 95–98% ee, together with the recovery of cyclopropanes 2c – e in good yields and with >90% ee (entries 2–4, Table 4 ). In contrast, electron-donating groups retarded the reaction. The reactions of 2f , g were run at 90 °C and gave adducts 5q , r with excellent ee values and obviously in lower yields. Cyclopropanes 2f , g were recovered with lower ee values (entries 5 and 6, Table 4 ). Oxindoles 2h – k with different donor groups (R 3 ) of the cyclopropane were also tried. As expected, with the R 3 group varying from the p -tolyl to phenyl and p -chlorophenyl groups, the reaction temperature increased from 50 to 60 and 70 °C (entry 1, Table 3 vs. entries 7–8, Table 4 ). The adducts 5s – v were all prepared satisfactorily. Cyclopropanes 2h – k were recovered in high yields and excellent ee values (entries 7–10, Table 4 ). Table 4 Scope of spirocyclopropyl oxindoles Full size table Notably, acetophenone-derived ketonitrones 9 are also viable substrates, enabling highly stereoselective synthesis of spirocylic oxindoles 10a – f with adjacent quaternary and tetrasubstituted carbon stereocenters (Fig. 3 ). It is worth mentioning that enantioselective catalytic reactions based on such unactivated achiral ketonitrones to create tetrasubstituted carbon stereocenters is unprecedented [65] , although two protocols using activated ketonitrones have been reported [66] , [67] . Fig. 3 Cycloaddition of spirocyclopropyl oxindoles using ketonitrones. Construction of adjacent quaternary and tetrasubstituted carbon stereocenters Full size image Proposed working model The relative configuration of racemic compound 4e and 5o was assigned by X-ray analysis. By converting to the corresponding N - p -tolylsulfonyl analogs, the relative and absolute configuration of compound 5a and 10a were also determined by X-ray analysis, as shown in Table 3 and Fig. 3 (for details, see Supplementary Figs. 1 and 2 ). Those of others were tentatively assigned by NMR analysis. Interestingly, no matter using N - p -tolylsulfonyl or N -diethoxyphosphoryl spirocyclic oxindoles, the cycloaddition reaction with nitrones afforded the major diastereomers of corresponding adducts in which the substituents at C3 and C6 of the tetrahydro-1,2-oxazine bore a trans relationship, different from the 3,6- cis selectivity of the known [3 + 3] cycloaddition of 2-substituted cyclopropane-1,1-dicarboxylates and nitrones [19] , [56] . The observed diastereoselectivity could be rationalized by the following working model involving a stepwise annulation mechanism (Fig. 4 ). According to previous studies in the Lewis acid catalyzed [3 + n] annulations of D–A cyclopropanes [21] , [58] , we proposed that the binding of the N -diethoxyphosphoryl oxindole 2 to the Lewis acid facilitated the O -attack of nitrones at the donor-substituted site of cyclopropane, leading to the reversion at that position, which was consistent with our experiments that under the catalysis of 10 mol% Ni(OTf) 2 , chiral cyclopropane (3 S , 8 R )- 2b with 90% ee afforded tetrahydro-1,2-oxazine (3 R , 4 R , 6 S )- 5m as the major product with 90% ee. The stepwise mechanism was also supported by the fact that the 1 H NMR analysis of the reaction mixture of nitrone 3a with N - p -tolylsulfonyl oxindole 1e could obviously detect the presence and the gradual disappearance of the intermediate correlating to the nucleophilic O -attack of nitrones to the donor-substituted site of cyclopropane (for details, see Supplementary Figs. 15 and 16 ). The resulting intermediate I further underwent an intramolecular Mannich cyclization to afford the desired product with 3,6- trans tetrahydro-1,2-oxazine, via a favored boat-like transition state IIa , which is possibly stabilized by the cation–π interaction between the iminium species and enolate [68] . The chiral-like transition state IIb , leading to the formation of 3,6- cis tetrahydro-1,2-oxazine, is presumably destabilized by the strong 1,3-diaxial repulsion between the N -methyl group of nitrone and the aromatic framework of oxindole. Fig. 4 Working model for the observed 3,6-trans selectivity of adducts 5 . A stepwise annulation mechanism. The favored boat-like transition state IIa is possibly stabilized by the cation–π interaction. The chiral-like transition state IIb is presumably destabilized by the strong 1,3-diaxial repulsion Full size image Synthetic application Impressively, our protocol provides a facile access to optically active oxindole-based spirocyclic tetrahydro-1,2-oxazines, and spirocyclopropyl oxindoles as well. It is noteworthy that optically active spirocyclopropyl oxindoles have wide application [33] . On the other hand, the N -diphenoxyphosphoryl group of adducts 5 could be readily removed, as evidenced by the conversion of 5a and 5o to the corresponding spirocyclic 1,2-oxazine 11a and 11b (Fig. 5 ). Fig. 5 Deprotection of product 5a and 5o . Reaction conditions: 5 (0.1 mmol), KOH (1.0 mmol) in 2.0 mL of EtOH at room temperature. Isolated yield Full size image In summary, we have demonstrated that spirocyclic oxindoles could be effectively activated by electron-withdrawing N -protecting group to serve as D−A cyclopropanes for complexity-generating synthesis. A highly enantioselective [3 + 3] cycloaddition and kinetic resolution of N -diethoxyphosphoryl spirocyclopropyl oxindoles is developed, providing a facile access to optically active oxindole-based spirocyclic tetrahydro-1,2-oxazines and spirocyclopropyl oxindoles of wide application [33] . This work also implies that catalytic enantioselective cycloaddition using spirocyclic D–A cyclopropanes is a promising approach for the flexible synthesis of chiral spirocyclic scaffolds. In addition, our work also suggests new synthetic opportunities of ketonitrones in creating tetrasubstituted carbon stereocenters. The evaluation of the biological activities of these spirocyclopropyl oxindoles is now in progress in our laboratories. The application of this strategy to explore other enantioselective cycloaddition additions is now under way in our laboratory. General methods See Supplementary Methods for further details. General procedure for catalytic enantioselective [3 + 3] cycloaddition of 2 and aldonitrone 3 To a Schlenk tube was sequentially added Ni(OTf) 2 (10.7 mg, 0.030 mmol, 10 mol%) and L 1 (11.8 mg, 0.033 mmol, 11 mol%), followed by the addition of anhydrous THF (3.0 ml). After the resulting solution was stirred at 50 °C for 2 h, oxindole 2 (0.30 mmol), nitrone 3 , and MS 3 Å (90 mg) were added successively. The reaction was kept stirring at the temperature indicated in Tables 3 and 4 till the full consumption of 3 by TLC analysis. Then THF was removed under reduced pressure. The residue was dissolved in CH 2 Cl 2 , rapidly passed through a glass funnel with a thin layer (5 mm) of silica gel (100 mesh), washed with CH 2 Cl 2 , and concentrated under reduced pressure. To determine the dr value of product, the residue was first dissolved in CDCl 3 , and took some samples to determine diastereoselectivity by 1 H NMR analysis. Then the sample for analysis and rest crude product were recombined for column chromatography purification to afford product 5 and recovered spirocyclopropyl oxindole 2 , using DCM/EtOAc (40/1, v/v) as the eluent. General procedure for catalytic enantioselective [3 + 3] cycloaddition of 2 and ketonitrone 9 To a Schlenk tube was sequentially added Ni(OTf) 2 (14.3 mg, 0.040 mmol) and L 1 (15.8 mg, 0.044 mmol), followed by the addition of anhydrous toluene (2.0 ml). After the resulting solution was stirred at room temperature for 2 h and cooled to 0 °C, nitrone 9 (0.2 mmol), oxindole 2 (0.44 mmol), and MS 3 Å (60 mg) were added successively. The reaction was kept stirring at 0 °C for 2 days. Then toluene was removed under reduced pressure. The residue was dissolved in CH 2 Cl 2 , rapidly passed through a glass funnel with a thin layer (5 mm) of silica gel (100 mesh), washed with CH 2 Cl 2 , and concentrated under reduced pressure. To determine the dr value of product, the residue was first dissolved in CDCl 3 , and took some samples to determine diastereoselectivity by 1 H NMR analysis. Then the sample for analysis and rest crude product were recombined for column chromatography purification to afford product 10 , using DCM/EtOAc (30/1, v/v) as the eluent. Data availability The X-ray crystallographic coordinates for structures reported in this study have been deposited at the Cambridge Crystallographic Data Centre (CCDC), under deposition numbers CCDC-1502102 (racemic major- 4e ), CCDC-1551103 (minor -4e ), CCDC-1502103 (major- 5o ) CCDC-1502104 ( 4e ), CCDC-1502105 ( 12a ), CCDC-1523864 ( 6 ), and CCDC-1523855 ( 8 ). These data can be obtained free of charge from The Cambridge Crystallographic Data Centre via www.ccdc.cam.ac.uk/data_request/cif . The authors declare that all other data supporting the findings of this study are available within the article and Supplementary Information files, and also are available from the corresponding author on reasonable request.